Pressure-induced semiconducting to metallic transition in multilayered molybdenum disulphide Molybdenum disulphide is a layered transition metal dichalcogenide that has recently raised considerable interest due to its unique semiconducting and opto-electronic properties. Although several theoretical studies have suggested an electronic phase transition in molybdenum disulphide, there has been a lack of experimental evidence. Here we report comprehensive studies on the pressure-dependent electronic, vibrational, optical and structural properties of multilayered molybdenum disulphide up to 35 GPa. Our experimental results reveal a structural lattice distortion followed by an electronic transition from a semiconducting to metallic state at ~19 GPa, which is confirmed by ab initio calculations. The metallization arises from the overlap of the valance and conduction bands owing to sulphur–sulphur interactions as the interlayer spacing reduces. The electronic transition affords modulation of the opto-electronic gain in molybdenum disulphide. This pressure-tuned behaviour can enable the development of novel devices with multiple phenomena involving the strong coupling of the mechanical, electrical and optical properties of layered nanomaterials. Recent advances in the preparation of atomically thin layers of van der Waals (vdW) bonded crystalline solids by mechanical exfoliation or chemical synthesis have allowed for renewed investigations of two-dimensional (2D) materials beyond graphene but with a similar layered hexagonal structure [1] , [2] , [3] , [4] , [5] . Within this class of 2D materials are transition metal dichalcogenides (TMDs), such as molybdenum disulphide (MoS 2 ), which have been increasingly explored to access a wealth of phenomena including opto-electronics [5] , valleytronics [6] , spintronics [7] and coupled electro-mechanics [8] . All of these phenomena arise from the complex thickness-dependent physical and electronic structures of the multilayered materials, in which the coupled electro-mechanics can be regarded as straintronics. Multilayered MoS 2 , having a band gap ( E g ) of ~1.2 eV [1] , is composed of stacked tri-atomic sheets where each tri-atomic monolayer exhibits a sandwiched structure with a plane of transition metal molybdenum atoms covalently bonded to, and sandwiched between, two planes of chalcogen sulphur atoms ( Fig. 1a ). Unlike monoatomic multilayered graphene with sp 2 hybridization, the diatomic composition of multilayered MoS 2 coupled with its d -orbital electronic states [9] and the small 6.5 Å vdW interlayer gap raises the prospects of strong sulphur–sulphur interlayer interactions under axial compression that might lead to an electronic phase transition. 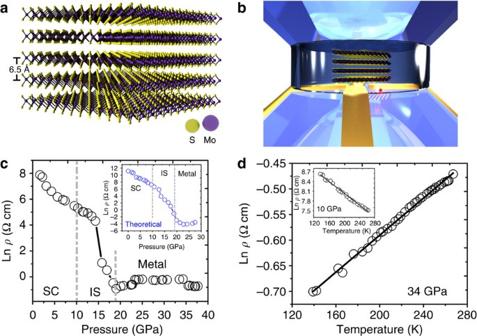Figure 1: Experimental setup and the electronic properties of multilayered MoS2. (a) The cross-section illustration of multilayered MoS2with an interlayer (caxis) spacing of ~6.5 Å. (b) A 3D illustration of multilayered MoS2in a DAC pressure medium for compression experiments. (c) Pressure-dependent electrical resistivity of MoS2. Three characteristic regions have been identified: semiconducting (SC), intermediate state (IS) and metallic regions. Inset: theoretically calculated pressure-dependent electrical resistivity. (d) Temperature-dependent resistivity of MoS2in the metallic state. Inset: the experimental temperature-dependent semiconducting behaviour of MoS2. The solid lines serve as visual guides. Figure 1: Experimental setup and the electronic properties of multilayered MoS 2. ( a ) The cross-section illustration of multilayered MoS 2 with an interlayer ( c axis) spacing of ~6.5 Å. ( b ) A 3D illustration of multilayered MoS 2 in a DAC pressure medium for compression experiments. ( c ) Pressure-dependent electrical resistivity of MoS 2 . Three characteristic regions have been identified: semiconducting (SC), intermediate state (IS) and metallic regions. Inset: theoretically calculated pressure-dependent electrical resistivity. ( d ) Temperature-dependent resistivity of MoS 2 in the metallic state. Inset: the experimental temperature-dependent semiconducting behaviour of MoS 2 . The solid lines serve as visual guides. Full size image Previously, several approaches have been undertaken to alter the solid-state properties of MoS 2 , including chemical doping [3] , [10] , [11] , [12] , intercalation [13] , [14] , surface functionalization [15] and defect engineering [11] , [16] , [17] . Furthermore, previous theoretical studies have suggested that an iso-structural semiconducting to metallic (S–M) transition in multilayered MoS 2 can be induced by pressure or strain [18] , [19] , [20] . Despite the broad interest in this phenomenon in layered nanomaterials, previous experimental results only reported a limited reduction in the electrical resistance [17] , [21] , [22] , [23] with no clear evidence for the pressure-induced S–M transition. In the present study, we have investigated high-purity exfoliated single crystalline MoS 2 with a stoichiometric chemical composition to evaluate the structural, vibrational, electrical and optical dependence at pressures up to 35 GPa. These results show a lattice distortion involving anisotropic c/a axial compression beginning at ~10 GPa in multilayered MoS 2 leading to an intermediate state (IS) followed by a pressure-induced S–M transition at ~19 GPa. First-principle theoretical calculations, which are performed to shed light on the underlying physics responsible for the S–M transition, attribute the origin of the metallic electronic states to sulphur–sulphur interactions as the vdW gap closes at high pressures. Our combined experimental and theoretical results here open a new window of opportunity for the development of nanoscale pressure switches, sensors and multi-physics devices with coupled electrical, vibrational, optical and structural properties using multilayered MoS 2 and semiconducting TMDs. Diamond anvil cell In this work, we have explored applied pressure effects via a high-pressure diamond anvil cell (DAC), as a controllable and reversible degree of freedom to modulate the properties of multilayered single-crystal MoS 2 . The DAC technique coupled with a hydrostatic pressure medium ( Fig. 1b ) has been shown to be effective in elucidating the electrical, vibrational, optical and structural properties of a plethora of materials [21] , [23] , [24] , [25] . The optically transparent window of the diamond allows us to conduct a series of in situ high-pressure experiments including accurate pressure calibration from ruby fluorescence, electrical transport measurements and optical Raman and synchrotron X-ray diffraction (XRD) spectroscopy [26] , leading to the observation of S–M transition in multilayered MoS 2 at high pressures. Pristine multilayered crystalline MoS 2 was transferred onto the DAC using micron-edged tweezers for investigations of the electronic, phononic and structural behaviours at pressures up to 35 GPa (see Methods for details). In addition, first-principle theoretical calculations were performed to elucidate the underlying material physics of the transition. Electrical conductivity and electronic structures In situ electrical conductivity measurements at room temperature using standard four-point metallic contacts reveal a gradual decrease in resistivity ( ρ ) with pressure up to 10 GPa, which can be understood in the context of a pressure-activated carrier transport model in good agreement with the experimental data (see Supplementary Note 1 and Supplementary Fig. 1 ). Between 10–19 GPa an abrupt decrease of about three orders of magnitude ( Fig. 1c ) is observed. Theoretical ab initio band structure calculations of the multilayer MoS 2 corroborates the experimental result with a predicted transition at ~20 GPa ( Fig. 1c , inset), which was theoretically found to correspond to a vanishing band gap owing to a S–M electronic transition. In addition, in situ temperature-dependent resistivity measurements were performed in the DAC in order to determine the resistivity profiles before and after the transition. It is well known from classical solid-state physics that resistivity decreases with temperature ( T ) for semiconductors owing to thermally activated carriers, in contrast to increasing resistivity for metallic conductors due to increased electron–phonon scattering [27] . Our resistivity measurements for multilayered MoS 2 reflect the aforementioned classical semiconducting behaviour as indicated by the negative temperature coefficient of resistivity at 10 GPa ( Fig. 1d , inset) for the semiconducting state, whereas a positive temperature coefficient of ρ is observed at 34 GPa for the metallic state ( Fig. 1d ). Moreover, the profile of the temperature-dependent resistivity magnitude shown in Fig. 1d follows an exponential decreasing trend at 10 GPa and a linear ( ρ α T ) trend at 34 GPa consistent with the classical behaviours of semiconducting and metallic materials respectively. Calculations using Boltzmann transport theory (BTT) for the temperature-dependent resistivity at ~10 GPa and 35 GPa support these experimental findings ( Supplementary Fig. 2 ). Furthermore, theoretical calculations determine that the semiconducting nature of MoS 2 originates from the fact that within a layer, Mo and S atoms are bound by mixed ionic and covalent bonding [28] . Under the application of pressure, the interlayer distance between the atomic planes decreases and the intra- as well as interlayer interactions are expected to alter the electronic properties of MoS 2 . Along the [0001] direction, MoS 2 with anisotropic linear incompressibilities will experience maximum compression, that is, the interlayer distance ( c axis) decreases more significantly than the intra-layer distance ( a axis). The hydrostatic pressure causes in- and out-of-plane strain. In order to analyse the effect of in-plane strain in achieving the S–M transition, we calculate the charge density redistribution keeping the in-plane strain constant, while varying the out-of-plane strain. 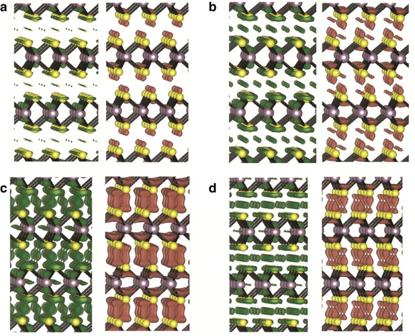Figure 2: Theoretical charge density isosurfaces of multilayered MoS2. Charge accumulation (green) and depletion (orange) at the (a) in-plane and out-of-plane strains of 2.2 and 6.9%, respectively, (b) in-plane and out-of-plane strains of 2.2 and 11%, respectively, and (c) in-plane and out-of-plane strains of 5.2 and 11%, respectively. (d) Same in-plane strain as in (c) but with 6.9% out-of-plane strain. Figure 2a,d shows the charge redistribution for a constant out-of-plane strain (6.9%) but at a different in-plane strain of 2.2 and 5.2%, respectively. Figure 2b,c shows the same but at a higher out-of-plane strain (11%). It can be seen that the interlayer interaction is enhanced with the increasing in-plane strain. Although, the S–M transition is caused by interlayer interaction due to the normal or out-of-plane strain, the in-plane strain helps to achieve this transition at a lower pressure. Figure 2: Theoretical charge density isosurfaces of multilayered MoS 2. Charge accumulation (green) and depletion (orange) at the ( a ) in-plane and out-of-plane strains of 2.2 and 6.9%, respectively, ( b ) in-plane and out-of-plane strains of 2.2 and 11%, respectively, and ( c ) in-plane and out-of-plane strains of 5.2 and 11%, respectively. ( d ) Same in-plane strain as in ( c ) but with 6.9% out-of-plane strain. Full size image With increasing pressure, our theoretical calculations show that the electronic charge moves away from the S atoms and accumulates onto the Mo atoms. Near the critical transition pressure, the maximum charge redistribution is predicted to occur in between the MoS 2 layers across the vdW gap, indicating enhanced S–S interaction. The change in the interlayer interaction from a weak vdW to a stronger interaction near the critical pressure is also supported by the derived lattice parameters using XRD spectra. However, these results do not give information regarding the orbitals involved in the charge transfer. Therefore, theoretical calculations for the angular momentum resolved density of states (LDOS) as a function of pressure were also performed to understand the contribution from the different orbitals of Mo and S atoms ( Supplementary Fig. 3 ). With increasing pressure, the contribution to the conduction band minima (CBM) from S- p x and S- p y orbitals decreases, while the contribution from S- p z orbitals increases. Similarly, there is a reduction with increasing pressure in contributions from Mo- p orbitals, while the contribution from Mo- d z 2 increases. Optical Raman vibrational spectroscopy Raman spectroscopy is considered to be a very accurate tool for gaining insight on the lattice vibrations of crystalline materials and has been commonly used to characterize the two prominent vibrational modes (E 2g and A 1g ) that are accessible in MoS 2 (refs 29 , 30 , 31 ). In order to elucidate the S–M electronic transition, Raman measurements were conducted in situ to probe vibrational changes in the multilayered MoS 2 under high pressure. It is well known that inducing pressure in MoS 2 results in an increase in the Raman shift ( Fig. 3a ) similar to other layered materials [30] , [32] . Analyses of the high-pressure Raman spectra reveal that the A 1g mode shows three distinct regions ( Fig. 3b ): (i) significantly increasing Raman shift up to about 10 GPa, (ii) nearly invariant shift with pressure between 10 GPa and 19 GPa and (iii) pressure-dependent Raman shift above 19 GPa. An evaluation of the Raman intensity ratio (between the E 2g and A 1g ) also reveals three distinct regions with the maximum intensity ratio observed in the metallic region ( Supplementary Fig. 4 ). We label these regions starting from low to high pressures as the semiconducting (SC), intermediate state (IS), and metallic regions respectively. In light of these observations, the out-of-plane vibrational mode (A 1g ) can be considered the more prominent Raman mode that is correlated with the semiconducting to metallic transition in MoS 2 , in contrast to the in-plane mode (E 2g mode) that shows a less distinct character across the transition. The IS can be understood within the context of phonon softening (PS), which describes the electron and A 1g phonon interaction where inter-valence charge transfer between the MoS 2 layers plays an important role in the structural distortion of the crystal symmetry [33] . Several materials have been previously reported to exhibit an intermediate state with soften phonon behaviour while undergoing a transition from a semiconductor to a metallic state [34] , [35] or when stress or strain is applied [36] , [37] . In fact, materials that exhibit superconductivity at high transition temperatures ( T c ) are often associated with structural distortions that are characterized by PS subsequently resulting in either a structural or electronic phase transition [38] . In our study here, the intermediate state ranges from ~10 GPa to 19 GPa where both the Raman shift for the A 1g mode ( Fig. 3b ) and the spacing between the two modes ( Fig. 3c ) show little dependence on pressure suggesting that the lattice structure is distorted. Moreover, the full-width at half-maximum (FWHM) of the two modes initially increases with pressure followed by a subsequent sharp drop of ~19 GPa ( Fig. 3d ). It should be noted that in a recent report, a drop in the FWHM was also observed during a phase transition in Sb 2 Se 3 , a topological insulator that exhibits a metallic state at the surface [39] . 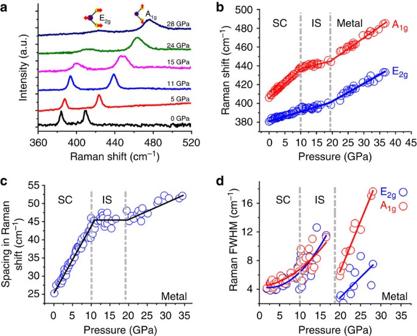Figure 3: Raman spectroscopic results of MoS2at high pressures. (a) Raman spectra at representative pressure points. The inset is an illustration of the in-plane and out-of-plane vibrations of the two key modes E2gand A1g, respectively. (b) The Raman shifts of the two modes with increasing pressures. The solid red and blue lines serve as visual guides. (c) The difference in Raman frequencies between the A1gand E2gmodes as a function of pressure flattens out in the IS state and rises at a smaller slope in the metallic region. The solid black line is a visual guide. (d) The FWHM for the A1gand E2gRaman modes across the electronic transition. A sharp drop is observed at ~19 GPa where MoS2transitions from the IS to a metallic phase. The solid red and blue lines serve as visual guides for the A1gand E2gmodes, respectively. Figure 3: Raman spectroscopic results of MoS 2 at high pressures. ( a ) Raman spectra at representative pressure points. The inset is an illustration of the in-plane and out-of-plane vibrations of the two key modes E 2g and A 1g , respectively. ( b ) The Raman shifts of the two modes with increasing pressures. The solid red and blue lines serve as visual guides. ( c ) The difference in Raman frequencies between the A 1g and E 2g modes as a function of pressure flattens out in the IS state and rises at a smaller slope in the metallic region. The solid black line is a visual guide. ( d ) The FWHM for the A 1g and E 2g Raman modes across the electronic transition. A sharp drop is observed at ~19 GPa where MoS 2 transitions from the IS to a metallic phase. The solid red and blue lines serve as visual guides for the A 1g and E 2g modes, respectively. Full size image The effect of pressure on the vibrational properties of MoS 2 can be further understood using theoretically calculated phonon dispersion curves based on the Perdew–Burke–Ernzerhof (PBE) functional method. We note that the calculated dispersion curves are consistent with that calculated using the local density approximation [26] , justifying the use of the method. Analysis of the A 1g and E 2g modes as a function of pressure (which can be identified at the calculated Γ point as shown in Supplementary Fig. 5 ) reveal that the splitting in the bands increases with applied pressure, resulting in significant changes in the Raman frequencies of the two modes ( Fig. 3b ). Opto-electronic properties Photoconductivity measurements have also been performed as a complementary means for understanding the opto-electronic properties of materials, which is dependent on the material’s band gap. To provide perspective, the pressure-dependent band gap for multilayered MoS 2 ( Fig. 4a ) can be understood from theoretical analysis using the PBE functional under the generalized gradient approximation (GGA). We note that the calculated unstrained E g of 1.03 eV is ~16% less than the experimental value [40] . This underestimation of the bandgap is a well-known problem due to the presence of artificial self-interaction and the absence of the derivative discontinuity in the exchange-correlation potential with the PBE/GGA methods [41] . Hybrid Heyd–Scuseria–Ernzerhof [42] functional and DFT with many-body perturbation theory in the GW approximation [43] are among the few methods to correctly predict the band gap of TMDs; however, these methods are computationally very expensive. Nevertheless, our previous study for bilayer MoS 2 has shown that the overall nature of the variation in the E g and the band structure with pressure are independent of the functional used [18] and that the PBE functional gives reasonably accurate results, justifying the use of the PBE/GGA methods for this work. With the increase in pressure, the degeneracy in the bands of the unstrained structure is lifted due to the enhanced interlayer interaction. The split bands in the valence band maxima (VBM) at the Γ point and the CBM between the K and Γ point start to move toward the Fermi level. The E g reduces consequently and becomes metallic when the CBM crosses the Fermi level at a pressure of 23.8 GPa ( Fig. 4a ), which correlates well with the transition pressures of ~19 GPa in the experimental resistivity measurements and Raman spectra. Analyses of the band structure in the metallic state indicate the overlap of the conduction and valence bands at the Fermi level ( Fig. 4b ). 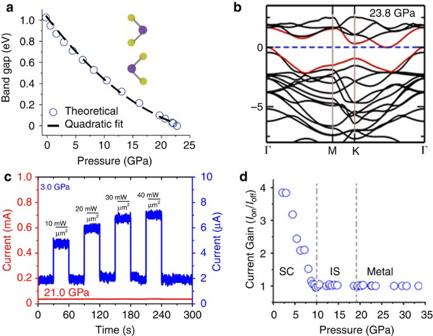Figure 4: Theoretical and experimental pressure-dependent opto-electronic properties of MoS2. (a) Theoretical calculation of the pressure-dependent band gap of multilayered MoS2. The bandgap—pressure dependence can be modelled as a quadratic function,Eg=Ego+aP+bP2was used, wherea=−70 meV GPa−1andb=1.13 meV GPa−2. Inset: the unit cell of MoS2. (b) Theoretical band structure of multilayered MoS2under hydrostatic pressure of 23.8 GPa. VBM and CBM are shown by red lines. (c) Optical switch behaviour before (blue lines at 3.0 GPa) and after (red line at 21.0 GPa) the S–M transition with various laser intensities. (d) Current gain (defined asIon/Ioffratio) as a function of pressure when exposed to a 532 nm (2.3 eV) laser light with an intensity of 40 W m−2. Figure 4: Theoretical and experimental pressure-dependent opto-electronic properties of MoS 2 . ( a ) Theoretical calculation of the pressure-dependent band gap of multilayered MoS 2 . The bandgap—pressure dependence can be modelled as a quadratic function, E g = E go + aP + bP 2 was used, where a =−70 meV GPa −1 and b =1.13 meV GPa −2 . Inset: the unit cell of MoS 2 . ( b ) Theoretical band structure of multilayered MoS 2 under hydrostatic pressure of 23.8 GPa. VBM and CBM are shown by red lines. ( c ) Optical switch behaviour before (blue lines at 3.0 GPa) and after (red line at 21.0 GPa) the S–M transition with various laser intensities. ( d ) Current gain (defined as I on / I off ratio) as a function of pressure when exposed to a 532 nm (2.3 eV) laser light with an intensity of 40 W m −2 . Full size image Unlike metals, semiconductors show an increase in the electrical conductivity when illuminated by light, and are therefore considered photoconductive. In particular, semiconducting MoS 2 has been found to offer sufficient photo-response that is suitable for practical photoconductive applications [3] , [4] , [5] , [44] . Opto-electronics require electron-hole generation/recombination, whereas the opto-electronic response of MoS 2 under green laser illumination (2.3 eV) in the event of a semiconducting to metallic transition in MoS 2 is expected to be significantly diminished in the metallic state ( Fig. 4c ). As a result, the photocurrent gain (ratio of current under illumination to dark current) was found to decrease with pressure as shown in Fig. 4d . The current gain decreases at a linear rate (Δ I gain /ΔGPa=−7.5%/GPa) until ~10 GPa where the current gain saturates to unity, indicating that photo-response is vanishing as the band gap begins to close. XRD and HR-TEM studies Electronic phase transitions can be accompanied by a structural or iso-structural phase transition. In order to clarify potential structural changes at high pressure, in situ high-pressure synchrotron XRD experiments were conducted to probe the perturbation of the crystal structure of multilayered MoS 2 under hydrostatic pressure. Two independent in situ high-pressure angle-dispersive XRD experimental runs were carried out at room temperature using a symmetric DAC. For the entire experimental pressure range, all the diffraction peaks can be refined to the hexagonal P6 3 /mmc structure using the Rietveld refinement [45] . On the basis of the hexagonal structure model, the crystal lattice parameters for MoS 2 from 0 to 28 GPa were calculated ( Fig. 5a ). The structure of the bulk unstrained MoS 2 can be viewed as ABAB stacked single layers of the material [22] . Though we did not observe any new peak(s) for multilayered MoS 2 up to 24 GPa in the XRD, a change along the c axis is observed at ~19 GPa, which suggests that the ambient lattice structure of MoS 2 is only weakly distorted. On the other hand, theoretical calculations were performed using the experimental lattice parameters as the reference, which are in close agreement with the GGA values. Results from theoretical pressure-dependent XRD calculations also confirm that there is no structural transition ( Supplementary Fig. 6 ). 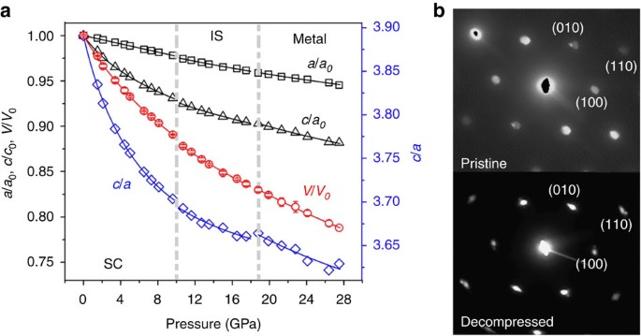Figure 5: Structural lattice parameters in multilayered MoS2. (a) Experimental pressure dependence of the lattice parameters of MoS2. The volume uncertainty bars are within 1% of the data. (b) The experimental SAED patterns of both pristine and decompressed MoS2. The patterns show that the single-crystal structure with the hexagonal symmetry was not significantly affected by high pressures and can be recovered back to its original crystal structure. Figure 5: Structural lattice parameters in multilayered MoS 2 . ( a ) Experimental pressure dependence of the lattice parameters of MoS 2 . The volume uncertainty bars are within 1% of the data. ( b ) The experimental SAED patterns of both pristine and decompressed MoS 2 . The patterns show that the single-crystal structure with the hexagonal symmetry was not significantly affected by high pressures and can be recovered back to its original crystal structure. Full size image Characterizing the atomic structure and quality of MoS 2 is critical for further understanding of the lattice distortion and electronic phase transition under pressure, and for ruling out the effects of lattice defects (that is, point defects, dislocations, grain boundaries and edges) that could play a role in influencing the experimental results [11] , [16] , [17] . For this purpose, high-resolution transmission electron microscopy (HR-TEM) and electron diffraction techniques were employed to evaluate the crystal structure of the same multilayered MoS 2 before and after the pressure loading experiments. The morphology of the starting sample in HR-TEM shows an atomic MoS 2 lattice having high crystallinity and the expected hexagonal lattice structure with a lattice spacing of 2.7 Å corresponding to the [100] direction ( Supplementary Fig. 7a ). The cross-section HR-TEM analysis shows the layered structure of MoS 2 having an interatomic c axis spacing of ~6.5 Å ( Supplementary Fig. 7b ). Transmission electron microscopy energy-dispersive X-ray spectroscopy (TEM-EDX) analyses were performed on both the pristine and decompressed MoS 2 to determine the stoichiometry, which was found to be a 1:2.07 ratio ( Supplementary Fig. 7c ), very close to the ideal 1:2 Mo:S ratio. Scanning electron microscopy (SEM) and scanning electron energy-dispersive X-ray spectroscopy (SEM-EDX) for both pristine and decompressed samples also show negligible difference ( Supplementary Fig. 7d ). The fast Fourier transformation (FFT) of the HR-TEM image shows the reflection spots from (100), (010) and (110), while the selected area electron diffraction (SAED) patterns for both the pristine and decompressed sample indicate the crystallinity and hexagonal symmetry were also unaffected by the applied pressures ( Fig. 5b ). The crystallographic results indicate that the starting sample was basically recoverable back to its original crystal structure. Collectively, the HR-TEM, TEM-EDX, FFT, SEM-EDX and SAED results indicate that the sample was of high crystalline quality and purity, and maintained its original chemical composition and lattice structure after the pressure-loading experiments. Previous studies have shown that loading of a crystal lattice via strain or hydrostatic pressure can cause a sharp reduction in resistivity, which is a precursor for an S–M transition [21] . In agreement with prior theoretical studies [18] , [19] , [46] , our theoretically predicted band gap is found to depend inversely on pressure and that the critical pressure for the electronic phase transition is predicted to scale down for multilayered films from ~16% normal compressive strain to ~11% for bilayer MoS 2 ( Supplementary Fig. 8 ). For monolayer MoS 2 this transition is predicted to occur at ~10% bi-axial strain [19] . Reported studies on other materials such as Sb 2 Te 3 (ref. 23 ), WSe 2 (ref. 24 ), BaNi 2 As 2 (ref. 38 ), FeS (ref. 47 ), V 2 O 3 (ref. 48 ) and VO 2 (ref. 49 ) have also shown a drop in resistivity before an electronic or structural phase transition in the material. These results have indicated that applying extremely high pressures onto such materials can even lead to a superconducting state. In MoS 2 , this drop in resistivity is correlated with the characteristic phonon modes (E 2g and A 1g ), and concurrent with phonon softening in the intermediate state, which has been observed as a precursor for resistivity transition in other materials [35] , [36] , [37] , [38] . We find that both the valence band (VB) and the conduction band (CB) originate from the Mo- d and S- p orbitals with the VB having minor contributions from the Mo- p orbital at zero pressure ( Supplementary Fig. 3 ). With increasing pressure, the contribution from the S- p z and Mo- d z 2 orbitals increases in both VB and CB, indicating a strong interlayer interaction. This analysis is in agreement with the charge redistribution. Experimentally, the bandgap can be extracted from temperature-dependent resistivity for intrinsic semiconductors; however, for the case of contemporary MoS 2 materials, the prevailing n-type character prevents bandgap extraction directly from resistivity data. We note that the A 1g mode arises from the out-of-plane vibration of the S atoms with enhanced S–S interactions as the vdW gap closes resulting in the observed metallization. In the intermediate state, vibrational phonon softening phenomenon in the Raman spectra has been studied extensively for other layered materials [39] , suggesting that it can be used as a clear signature for the electronic phase transition in the multilayered MoS 2 . The pressure-dependent Raman frequency increase was observed to be higher for the out-of-plane A 1g mode than that of the in-plane E 2g mode. This clearly indicates an enhancement of interlayer interactions with pressure. The multitude of pressure-dependent Raman spectra characteristics (FHWM, intensity ratio and peak spacing) are well correlated with the pressure-dependent resistivity, all showing an abrupt or particular response in the IS region. These strong correlations provide unambiguous experimental and theoretical support for the semiconducting to metallic phase transition in multilayered MoS 2 . Since the neighbouring planes of the sulphur atoms along the c axis are bonded by weak vdW forces, the c axis contracts two times more than the a axis below 28 GPa, exhibiting strong anisotropic compressional properties. The c / a lattice-parameter ratio decreases monotonically with pressure up to 19 GPa, which indicates that the interactions between the adjacent planes of sulphur atoms become stronger under pressure. We note that the c / a curve profile shows discontinuity at ~19 GPa. Similar behaviour was also reported by Aksoy et al. [50] and can be attributed to a pressure-induced structural distortion in which MoS 2 layers slide from the original 2H c -MoS 2 to the 2H a -MoS 2 structure [24] . Based on theoretical studies by Hromadová et al. [22] , the peak positions in Raman measurements under high pressure coincide with the electronic properties of the emergent 2H a -MoS 2 phase. We thus conclude that the observed changes in the electrical and vibrational response can be solely attributed to an iso-structural electronic phase transition. We have demonstrated for the first time that a drastic drop in resistivity can be attributed to an electronic phase transition from semiconducting to metallic in multilayered MoS 2 , which is further corroborated by in situ temperature-dependent resistivity measurement and Raman spectroscopy. Our results can be applied to novel MoS 2 devices, where pressure can be an external stimulus to dynamically control the band gap and tune the opto-electronic response or photoconductive gain. The experimentally observed transition is in good agreement with ab initio theoretical calculations, allowing one to predict the thickness dependence of the critical transition pressure. Based on the similarity in the crystal and band structure of the semiconducting transitional metal dichalcogenides, the observed electronic phase transition in MoS 2 is likely to be experimentally accessible in MoSe 2 , WS 2 and WSe 2 as predicted in a previous work [18] . The combined experimental results and theoretical insights indicate a new opportunity for the development of multi-physics device concepts with coupled mechanical, electrical and optical properties based on the tunable and unique material structure of the semiconducting transitional metal dichalcogenides. Sample characterization MoS 2 single crystals were purchased from SPI Supplies (CAS# 1317-33-5). The purity of the crystals was characterized and estimated to be >99% by SPI supplies. The crystals were then thinned down to flakes of ~150 nm thick and 100 μm in length. Cross-section HR-TEM analyses of the sample flakes showed chemically and physically homogeneous layer surfaces at the nanometre scale. To understand the characteristics of the pristine as well as pressure-quenched samples (up to ~35 GPa and then quenched to ambient pressure), HR-TEM was used to analyse the lattice structures at the nanometre scale. Pristine MoS 2 was exfoliated onto a Cu TEM grid (SPI# 2040C-XA), while the quenched MoS 2 was transferred onto the Cu TEM grid using a micro tip-needle for HR-TEM analyses. The beam spot size was 5 nm in the TEM-EDX and an aperture size of 160 nm was used for the selected area electron diffraction (SAED). HR-TEM analyses of the recovered samples from DAC compression experiments show that their crystallinity and hexagonal lattice structure have not been altered drastically by compression and decompression in the DAC ( Fig. 5 and Supplementary Fig. 7 ). High-pressure electrical resistance measurements Four-point probe electrical technique was employed to measure the electrical resistivity of the single-crystal multilayered MoS 2 as a function of pressure. Resistivity measurements as a function of temperature were also conducted in the SC, IS and metallic state. A modified short symmetric DAC having a pair of anvil culets of 400 μm or 500 μm was used in two separate runs to ensure reproducibility. A rhenium gasket was pre-indented from a thickness of 250 μm to 40 μm at ~20 GPa, and a hole with a diameter of 200 μm was drilled in the centre of the pre-indented area. Cubic BN (c-BN) fine powders were used as an insulating layer that was pressed into the pre-indented area and the drilled hole. Consequently, another hole of 100 μm in diameter was drilled at the centre of the 200 μm hole filled with c-BN, which was then further filled with soft h-BN fine powders as the pressure-transmitting medium while neon was used as the gas medium. A MoS 2 single crystal of 150 nm thick with dimensions of ~100 μm × 266 μm was loaded into the sample chamber, together with three ruby spheres as the pressure calibrant and four Au electrodes with a length of 12.5 μm for EC measurements. The resistivity of the sample was obtained by measuring the DC current changes in a pair of Au probes while sweeping DC voltages in another pair. The sample resistivity was derived by measuring the slope of the current–voltage ( I – V ) plot after taking the sample thickness into account [51] . Quenched samples were further examined using cross-sectional SEM for potential dimensional changes of the samples to ensure reliable EC correction. For the opto-electronic measurements under high pressure, a green laser with 532 nm wavelength (2.3 eV) was focused down to a 10 μm × 10 μm window to ensure that the laser was exclusively on the sample. High-pressure laser Raman spectroscopy Raman spectra were measured using a green 532 nm Coherent Verdi V2 laser. The scattered light was dispersed by a 1,800 groves per mm grating and collected by an EMCCD (Andor Technology) resulting in a spectral resolution of ~1 cm −1 . The highest laser power level of 4 mW with a focused laser beam size of 10 μm was used for the measurements to avoid potential over-heating or oxidation of the samples. Ruby fluorescence spectra were also collected using the same system for pressure calibrations; pressures and their uncertainties were determined from multiple measurements of the ruby spheres close to the sample in the sample chamber of the DAC before and after each Raman measurement. High-pressure synchrotron XRD experiments In situ high-pressure angle-dispersive XRD experiments were carried out at the High Pressure Collaborative Access Team (HPCAT) and GeoSoilEnviroCARS (GSECARS) of the Advanced Photon Source (APS), Argonne National Laboratory using a wavelength of 0.4066 Å and 0.3344 Å, respectively, in a symmetric DAC. The diameter of the diamond culets was 400 μm while the thickness of the sample loaded into the sample chamber was ~20–25 μm. A Rhenium gasket pre-indented to 45 μm thick with a drilled hole of 150 μm in diameter was used as the sample chamber, while neon was used as the pressure-transmitting medium and the pressure was measured using a ruby fluorescence calibrant. XRD images were collected by an MAR CCD and were integrated using the Fit2D programme [52] . The integrated XRD patterns were further analysed using the GSAS programme package for the Rietveld refinement [45] . The solid line is the fitting result ( Fig. 5a ) using the third-order Birch–Murnaghan equation of state (BM EoS) [53] , [54] : where V and V 0 represent the high-pressure and ambient-pressure unit cell volume, respectively; K 0 and refer to the bulk modulus and its pressure derivate at ambient conditions, respectively. The isothermal bulk modulus K 0 for the semiconducting state, IS state, and the metallic state was derived to be 57 GPa, 51 GPa and 64 GPa wih being 4.6 GPa, 4.9 GPa and 4.2 GPa respectively. First-principle theoretical calculations Theoretical calculations were carried out using first-principle ab initio DFT using Vienna Ab initio Simulation Package (VASP) [55] . All-electron projector augmented wave potentials [56] , [57] and the PBE [58] GGA were used to account for the electronic exchange and correlation. The weak vdW interaction was incorporated by adding a semi-empirical dispersion potential (D) to the conventional Kohn–Sham DFT energy, through a pair-wise force field following Grimmes DFT-D2 method [59] . The crystal structure was optimized by employing a conjugate gradient scheme until the forces on every atom were minimized to be <0.005 eV Å −1 , and that a well-converged Monkhorst–Pack k -point set (17 × 17 × 6) was used for this procedure. The phonon dispersion of MoS 2 was calculated using density functional perturbation theory [60] as implemented in VASP. An additional tool, Phonopy [61] , which supports the VASP interface, was used for extracting the phonon frequencies. The force-constants were calculated with a supercell of 2 × 2 × 2 and the k -point set of 9 × 9 × 3. The criterion for the force convergence used for the phonon calculations was 10 −8 eV Å −1 . Electrical conductivity of MoS 2 is calculated using BTT within the constant scattering time approximation (CSTA) [27] , [62] , as implemented in the BoltzTraP programme [63] . In the CSTA, it is assumed that the scattering time ( τ ) determining the electrical conductivity does not vary strongly with temperature. In the BTT, the motion of an electron is treated semi-classically. The group velocity of an electron in a particular band can be described as: Where ε( i , k ) is the i th energy band at point k and k α is αth component of wave-vector k . From the group velocity v α ( i , k ), the electrical conductivity tensor can then be calculated by the following equation: where τ( i , k ) is the relaxation time, α and β are the Cartesian indices, N is the total number of k -points sampled, V is the volume of the unit cell, f μ is the Fermi Dirac distribution function and e is the elementary charge. In order to estimate the electrical transport properties of bulk MoS 2 , first the calculations for the electronic structure were performed using a denser k -point set of 32 × 32 × 8. This was followed by the calculation of group velocities by Fourier interpolation [64] of the band energies as a function of k . Consequently, the transport properties were calculated by using equation (3). From the electronic structure it is possible to calculate σ / τ as a function of temperature ( T ) and carrier concentration ( n ), but it is not possible to calculate σ without relaxation time ( τ ). To approximate the relaxation time, we used experimental data from Mahalaway et al. [65] The reported experimental electrical conductivity is 0.03 Ω −1 cm −1 at room temperature, which combined with the calculated σ / τ yield τ =7.5 × 10 −14 . We then calculate σ as σ / τ × τ . How to cite this article: Nayak, A. P. et al. Pressure-induced semiconducting to metallic transition in multilayered molybdenum disulphide. Nat. Commun. 5:3731 doi: 10.1038/ncomms4731 (2014).